Intron retention in theDrosophila melanogaster Rieske iron sulphur proteingene generated a new protein Genomes can encode a variety of proteins with unrelated architectures and activities. It is known that protein-coding genes of de novo origin have significantly contributed to this diversity. However, the molecular mechanisms and evolutionary processes behind these originations are still poorly understood. Here we show that the last 102 codons of a novel gene, Noble , assembled directly from non-coding DNA following an intronic deletion that induced alternative intron retention at the Drosophila melanogaster Rieske Iron Sulphur Protein ( RFeSP ) locus. A systematic analysis of the evolutionary processes behind the origin of Noble showed that its emergence was strongly biased by natural selection on and around the RFeSP locus. Noble mRNA is shown to encode a bona fide protein that lacks an iron sulphur domain and localizes to mitochondria. Together, these results demonstrate the generation of a novel protein at a naturally selected site. Natural selection and neutral drift have been postulated to shape de novo coding sequences following their assembly from non-coding DNA [1] , [2] , [3] . However, the processes, or constraints, that lead to the origin of novel coding regions have seldom been studied systematically. This might be because, despite recent advances in genome sequencing, it remains a challenge to reconstruct with confidence the evolutionary pathway of the origination of any novel coding region [1] , [2] , [3] , [4] , [5] . Random genetic drift, population bottlenecks, genetic sweeps and the extinction of species are a few of the natural processes that affect the frequency of transitional alleles and commonly contribute to a discontinuous mutational lineage through time. Fortunately, decades of theoretical work on the neutral theories of evolution as a null hypothesis for molecular evolution [6] , [7] , [8] , [9] have provided a solid theoretical framework for understanding gene origination. This work also allows us to test whether any de novo gene origination would arise as a consequence of non-adaptive mechanisms by the stochastic accumulation of neutral or quasi-neutral mutations. Rieske iron sulphur proteins (RFeSPs) are essential, highly conserved functional constituents of energy-transducing respiratory complexes [10] . Drosophila melanogaster is predicted to have a complex RFeSP locus encoding at least two different proteins by an alternative intron-retention mechanism, according to published reference sequences [11] , [12] , [13] , [14] ( Fig. 1a ). Briefly, the conserved RFeSP isoform (annotated as RFeSP-PB) is encoded by the RFeSP-RB transcript, which arises following splicing of the second intron of the locus (hereafter referred to as intron2 ). An alternative transcript, RFeSP-RA , forms following intron2 retention, which shifts the reading frame of the 3′-end of the gene. The resulting RFeSP-PA protein is predicted to contain 102 amino acids (aa) of novel sequence at its carboxy (C)-terminus instead of the last 72 aa of the C-terminal iron-sulphur cluster-binding domain found in RFeSP-PB ( Fig. 1a ). 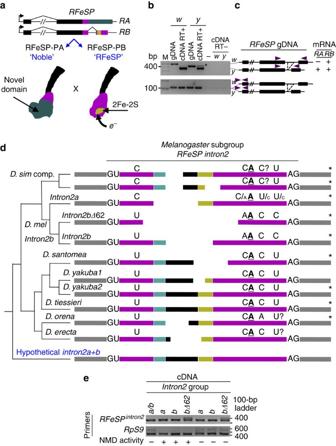Figure 1: TheD. melanogaster RFeSPlocus encodes a novel transcript by alternative intron retention. (a) The alternatively spliced transcriptsRFeSP-RAand -RBencode a novel 260-aa protein (RFeSP-PA; herein renamed Noble) and the conserved 230-aa RFeSP protein (RFeSP-PB;akaRFeSP), respectively. Both share the first 158 aa, which contain the ubiquinol cytochrome reductase transmembrane region (black) and part of the Rieske domain (magenta; aa K107to D158). Retention ofintron2then shifts the reading frame inRFeSP-RAgenerating ade novodomain in RFeSP-PA instead of the [2Fe-2S] cluster-binding domain that mediates electron transfer in the mitochondria. (b) Agarose gel of PCR and RT–PCR products. Lane 1: 100-bp DNA ladder (M); lane 2:w1118(w) genomic DNA (gDNA); lane 3:wRT+ cDNA; lane 4: genome reference strain (y) gDNA; lane 5:yRT+ cDNA; lane 6: dH2O; lane 7:wRT– cDNA; lane 8:yRT– cDNA. Asterisk denotesRFeSP-RAtranscript. (c) Association between theRFeSP-RAmRNA and a deletion within theRFeSP intron2from theygenome reference strain. Magenta arrowheads: position of primers used inb. (d) Gene phylogeny (not to scale) of theRFeSP intron2. Cyan and dark yellow bars: mutually exclusive sequences (10 and 8-bp, respectively), which characterizeintron2aandintron2bgroups, respectively, inD. melanogaster (D. mel)or homologous sequences in other species. Black bars: other homologous stretches. Grey sequences: exonic RNA. Magenta bars: the rest ofintron2. GU and AG: intron donor and acceptor, respectively. Key polymorphic nucleotides are shown. The branch point 'A' is underlined. '?' Depicts uncertain nucleotides. Underscript: putative recombinants,n=2/26 forintron2a.Intron2a+b: hypothetical ancestralintron2.D. sim: D. simulans. Asterisks indicate taxa sequenced in our study. (e) Agarose gel showing RT–PCR products from NMD-susceptible regions ofRFeSP intron2and RpS9 (control). Lane 1:intron2group genotype:intron2a/intron2b(a/b;heterozygote), strainUpf125G(NMD activity negative (−)); lane 2:intron2agenotype (a), strainw1118(NMD+); lane 3:intron2bgenotype (b), strain Samarkland (NMD+);intron2bΔ62genotype (bΔ62), strain Canton-S (NMD+); lane 5–7, sameintron2genotypes as lanes 2–4, respectively, but in aUpf125GNMD-hemyzygote background. Figure 1: The D. melanogaster RFeSP locus encodes a novel transcript by alternative intron retention. ( a ) The alternatively spliced transcripts RFeSP-RA and - RB encode a novel 260-aa protein (RFeSP-PA; herein renamed Noble) and the conserved 230-aa RFeSP protein (RFeSP-PB; aka RFeSP), respectively. Both share the first 158 aa, which contain the ubiquinol cytochrome reductase transmembrane region (black) and part of the Rieske domain (magenta; aa K 107 to D 158 ). Retention of intron2 then shifts the reading frame in RFeSP-RA generating a de novo domain in RFeSP-PA instead of the [2Fe-2S] cluster-binding domain that mediates electron transfer in the mitochondria. ( b ) Agarose gel of PCR and RT–PCR products. Lane 1: 100-bp DNA ladder (M); lane 2: w 1118 ( w ) genomic DNA (gDNA); lane 3: w RT+ cDNA; lane 4: genome reference strain ( y ) gDNA; lane 5: y RT+ cDNA; lane 6: dH 2 O; lane 7: w RT– cDNA; lane 8: y RT– cDNA. Asterisk denotes RFeSP-RA transcript. ( c ) Association between the RFeSP-RA mRNA and a deletion within the RFeSP intron2 from the y genome reference strain. Magenta arrowheads: position of primers used in b . ( d ) Gene phylogeny (not to scale) of the RFeSP intron2 . Cyan and dark yellow bars: mutually exclusive sequences (10 and 8-bp, respectively), which characterize intron2a and intron2b groups, respectively, in D. melanogaster (D. mel) or homologous sequences in other species. Black bars: other homologous stretches. Grey sequences: exonic RNA. Magenta bars: the rest of intron2 . GU and AG: intron donor and acceptor, respectively. Key polymorphic nucleotides are shown. The branch point 'A' is underlined. '?' Depicts uncertain nucleotides. Underscript: putative recombinants, n =2/26 for intron2a . Intron2a+b : hypothetical ancestral intron2 . D. sim: D. simulans . Asterisks indicate taxa sequenced in our study. ( e ) Agarose gel showing RT–PCR products from NMD-susceptible regions of RFeSP intron2 and RpS9 (control). Lane 1: intron2 group genotype: intron2a/intron2b ( a/b; heterozygote), strain Upf1 25G (NMD activity negative (−)); lane 2: intron2a genotype ( a ), strain w 1118 (NMD + ); lane 3: intron2b genotype ( b ), strain Samarkland (NMD + ); intron2b Δ 62 genotype ( b Δ 62 ), strain Canton-S (NMD + ); lane 5–7, same intron2 genotypes as lanes 2–4, respectively, but in a Upf1 25G NMD-hemyzygote background. Full size image Here, the evolutionary history of RFeSP-PA was systematically investigated, and both the neutrality and stochasticity of its origin were tested. We found out that the last 102 codons of RFeSP-RA assembled de novo from non-coding DNA in a single step after a nearly neutral intronic deletion caused the alternative retention of the second intron of the RFeSP-RB gene. Analyses of the evolutionary processes affecting the RFeSP locus before the emergence of RFeSP-RA then allowed us to determine and dissect the role played by natural selection as a significant source of bias affecting the origination of RFeSP-RA . RFeSP-RA is associated with a polymorphic intronic deletion To confirm the annotated prediction that the D. melanogaster RFeSP locus encodes two isoforms, reverse transcriptase (RT)–PCR was performed to amplify across intron2 using cDNAs from two different standard fly stocks ( Fig. 1b ). Both the novel RFeSP-RA and the conserved RFeSP-RB isoforms are produced in the Berkeley Drosophila Reference Sequencing Strain [11] , [12] (reference genome strain y 1 ; cn 1 bw 1 sp 1 ). However, even though total RFeSP transcript levels were similar, no RFeSP-RA was detectable in another standard strain w 1118 ( Fig. 1b ). To test whether the alternative splicing of RFeSP was associated with any underlying genetic alteration, PCR was performed using genomic DNA isolated from both w 1118 and the reference genome strains. The reference genome strain carried an ∼ 50-bp shorter intron2 than the w 1118 strain ( Fig. 1b,c ). These experiments showed that RFeSP-RA expression was associated with a variation in intron2 length ( Fig. 1c ). Single-step assembly of 102 de novo codons of RFeSP-RA To discover the origin and frequency of the intron2 variants that produce the novel RFeSP-RA transcript, ∼ 300 bp of DNA sequence spanning intron2 were obtained from 57 lines of D. melanogaster of geographically diverse origin, as well as from a series of lines from closely related Drosophila species ( Supplementary Table S1 ). The sequences were aligned by hand and clustered into haplotypes ( Supplementary Fig. S1 ). Results suggested that the RFeSP-RA -productive intron2 variant of the reference genome strain was identical to, and most likely originated from, the Canton-S wild-type stock. The number of strains with this short Canton-S-like intron2 haplotype was low compared with the number of strains with the longer intron2 variants, which were most similar in length to the w 1118 intron2 allele ( Supplementary Fig. S1 ). These longer intron2 sequences clustered into two major allelic groups hereafter named as intron2a and intron2b , which are 115 and 117 bp in size, respectively ( Fig. 1d and Supplementary Fig. S1 ). Using phylogenetically informative single-nucleotide polymorphisms within intron2 , we determined that an intron2b allele directly gave rise to the RFeSP-RA -productive intron2 allele found in Canton-S by a 62-bp deletion ( Fig. 1d ); hence, the latter was named intron2b Δ 62 . This finding raised the possibility that the deletion intron2b Δ 62 directly caused the emergence of RFeSP-RA mRNA and the generation of the last 102 codons of RFeSP-RA in a single step. Supporting this interpretation, we found that no RFeSP-RA -like mRNA was detectable by RT–PCR in a strain carrying the intron2b genotype directly ancestral to intron2b Δ 62 ( Fig. 1e ). Furthermore, no RFeSP-RA cDNA could be detected by RT–PCR in a nonsense-mediated decay (NMD) [15] , [16] defective background carrying the ancestral intron2b allele ( Fig. 1e ). This indicated that in the ancestral intron2b allele, an RFeSP-RA -like mRNA is not being generated and then degraded by NMD. These results strongly suggest that the intron2b Δ 62 deletion itself was the cause of the de novo RFeSP-RA mRNA emergence. A plausible mechanism to explain the facultative intron2 retention is that the putative branch point is positioned only 31 bp downstream of the 5′ splice donor in intron2b Δ 62 , ( Fig. 1d ; Supplementary Fig. S1 ). This distance is shorter than the ∼ 38-bp limit found between the 5′ splice donor and the branch point in previous D. melanogaster intron-sequence analyses [17] . In the alleles that are efficiently spliced, the predicted branch points are longer than the 38-bp limit. Together, these data suggest that the intron2b Δ 62 deletion directly caused the emergence of the RFeSP-RA mRNA by creating a suboptimal distance between the 5′ splice donor and the branch point in this allele (that is, intron recognition is poor, but still possible), giving rise to inefficient splicing of this intron. Given that RFeSP is an essential gene [18] , Canton-S flies might have survived and/or fixed intron2b Δ 62 because it still allowed production of the canonical RFeSP protein, albeit less efficiently. Nonneutral evolution of RFeSP intron2 alleles To determine the mutational events, as well as the selective pressures that allowed the intron2b Δ 62 deletion, the recent evolutionary history of its immediately ancestral allele, intron2b , was investigated. Molecular phylogenetic analyses indicate that virtually no intronic sequence gain has taken place and/or has become fixed in the melanogaster subgroup for 6–12 million years (MYs) [19] , [20] (see Fig. 1d ). Instead, several deletions occurred in intron2 during melanogaster subgroup speciation. Phylogenetic analyses of the deletions showed that they could be treated as irreversible shared derived cladistic characters [21] . Cladistic parsimony implies that the D. melanogaster intron2a and intron2b groups could not have originated from each other and that they must have originated independently from a 'complete' intron2a+b ( Fig. 1d ). Although sequencing efforts failed to find such intron2a+b segregating in D. melanogaster , even in sub-Saharan populations where this species originated [22] , [23] , many examples of intron2a+b -like introns were found in other melanogaster subgroup species, allowing us to devise the likely overall structure of the melanogaster subgroup intron2 ancestor ( Fig. 1d ). From this molecular phylogeny, it was concluded that the intron2a and intron2b groups are ancient and their existence as allelic groups either precedes, or coincides, with D. melanogaster speciation. As the ancient nature of intron2 allele groups could have important implications for the understanding of the evolutionary processes that acted on RFeSP before the emergence of RFeSP-RA , the RFeSP locus was investigated further using a population genetics perspective. We found that RFeSP intron2b alleles had strikingly less nucleotide diversity than intron2a , and, although neutrality tests were generally nonsignificant when all intron2 alleles were considered together, when analysed separately the neutral hypothesis was rejected in three out of four neutrality tests for the intron2b group alleles, while none were rejected for intron2a ( Fig. 2a ; Supplementary Table S2 ). Furthermore, a difference between intron2 groups was also evident when the average ratio between nonsynonymous and synonymous substitution rates (d N /d S ) on the coding regions of each group was calculated, revealing a complete absence of nucleotide substitution in the coding regions of intron2b group alleles [21] , [24] ( Supplementary Fig. S2 ). Two conclusions were drawn from these results about the evolution of the intron2b group: first, it deviated from that expected from neutrally drifting alleles, and second, it deviated from what one would expect if it were as ancient as the intron2a group. As intron2b is the ancestral allele of intron2b Δ 62 , these findings demonstrate that RFeSP-RA emerged from skewed nucleotide sequences. 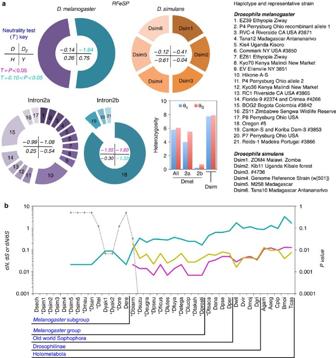Figure 2: Nonneutral evolution ofintron2binD. melanogaster. (a) Donut-shaped frequency charts of majorD. melanogaster RFeSP intron2groups. Haplotype frequency for each majorD. melanogaster intron2group (aorb, in cyan and purple, respectively) is shown separately below. Haplotypes are numbered according to the list on the right side.D. simulans RFeSP intron2haplotype frequency chart also shown as a reference (orange). Neutrality tests (T) results are shown according to key. D=Tajima's D, D2=Fu and Li's D2, H=Fay and Wu's H, and Y=Achaz's Y. A statistically significantTvalue is depicted in red. θSand θπare heterozygosity (nucleotide diversity) indicators. (b) Left axis: ratios of nonsynonymous (dN, magenta line) to synonymous substitutions (dS, cyan line), and their rate (dN/dS, dark yellow line) between a 191-bpRFeSP-coding fragment fromD. melanogasterand different taxa. Right axis: Fischer's exact testPvalues (dashed grey line).D. sechellia(Dsech),D. simulans(Dsim1–6),D. mauritiana(Dmau),D. yakuba(Dyak1–2),D. teissieri(Dtei),D. erecta(Dere),D. orena(Dore), D.santomea(Dsan),D. biarmipes(Dbiarm),D. suzukii(Dsuzu),D. eugracilis(Deugra),D. pseudotakahashii(Dpseu),D. ficusphila(Dficus),D. lutescens(Dlutes),D. fuyamai(Dfuya),D. elegans(Delega),D. lucipennis(Dlucip),D. takahashii(Dtakah),D. prostipennis(Dprosti),D. tsacasi(Dtsaca),D. ananassae(Dana),D. pseudoobscura(Dpse),D. persimilis(Dper),D. willistoni(Dwil),D. virilis(Dvir),D. mojavensis(Dmoj),D. grimshawi(Dgri),Anopheles gambiae(Agam),Aedes aegypti(Aaeg),Culex pipiens(Cpip),Bombyx mori(Bmor) andTribolium castaneum(Tcas). Asterisks indicate taxa sequenced in this study. Figure 2: Nonneutral evolution of intron2b in D. melanogaster . ( a ) Donut-shaped frequency charts of major D. melanogaster RFeSP intron2 groups. Haplotype frequency for each major D. melanogaster intron2 group ( a or b , in cyan and purple, respectively) is shown separately below. Haplotypes are numbered according to the list on the right side. D. simulans RFeSP intron2 haplotype frequency chart also shown as a reference (orange). Neutrality tests ( T ) results are shown according to key. D=Tajima's D, D 2 =Fu and Li's D 2 , H=Fay and Wu's H, and Y=Achaz's Y. A statistically significant T value is depicted in red. θ S and θ π are heterozygosity (nucleotide diversity) indicators. ( b ) Left axis: ratios of nonsynonymous (d N , magenta line) to synonymous substitutions (d S , cyan line), and their rate (d N /d S , dark yellow line) between a 191-bp RFeSP -coding fragment from D. melanogaster and different taxa. Right axis: Fischer's exact test P values (dashed grey line). D. sechellia (Dsech), D. simulans (Dsim1–6), D. mauritiana (Dmau), D. yakuba (Dyak1–2), D. teissieri (Dtei), D. erecta (Dere), D. orena (Dore), D. santomea (Dsan), D. biarmipes (Dbiarm), D. suzukii (Dsuzu), D. eugracilis (Deugra), D. pseudotakahashii (Dpseu), D. ficusphila (Dficus), D. lutescens (Dlutes), D. fuyamai (Dfuya), D. elegans (Delega), D. lucipennis (Dlucip), D. takahashii (Dtakah), D. prostipennis (Dprosti), D. tsacasi (Dtsaca), D. ananassae (Dana), D. pseudoobscura (Dpse), D. persimilis (Dper), D. willistoni (Dwil), D. virilis (Dvir), D. mojavensis (Dmoj), D. grimshawi (Dgri), Anopheles gambiae (Agam), Aedes aegypti (Aaeg), Culex pipiens (Cpip), Bombyx mori (Bmor) and Tribolium castaneum (Tcas). Asterisks indicate taxa sequenced in this study. Full size image To distinguish the mechanism for the reduced polymorphisms found in intron2b , we carried out linkage disequilibrium analyses between RFeSP intron2 groups and two possible proximal sites previously described to have been associated with positive selection [25] , [26] ( Supplementary Figs S3 and S4 ). Results showed that gene-copy polymorphisms in the tightly linked ( ∼ 0.2 cM) Odorant receptor 22 ( Or22 ) locus could significantly explain a large fraction of intermediate (a subset of intron2a ) and high-frequency (all alleles from intron2b ) RFeSP haplotypes ( Supplementary Fig. S4 ). These analyses suggested that, apart from population history, positive selection could account for both the dip in nucleotide diversity in all high-frequency alleles, as well as for the linkage disequilibrium between them and variation at the Or22 locus ( Supplementary Fig. S4 ). These findings warrant further study by using Chr2 isochromosomal lines and sequencing of multiple adjacent loci to probe further into this association. RFeSP-RA codons were biased by negative selection on RFeSP To further study the possible effect of selection on the nucleotide sequence that eventually became part of RFeSP-RA , the earliest time since when this exact RFeSP locus has been under selective pressure was determined. d N /d S ratios were generally not measurable between melanogaster subgroup species, because there were virtually no nonsynonymous changes in the surveyed sequences ( Fig. 2b ). Albeit synonymous changes occurred, they were underrepresented. For instance, only 29.6% (8/27) and 22.2% (4/18) of the segregating polymorphisms found for D. melanogaster and D. simulans , respectively, were synonymous changes ( Supplementary Fig. S1 ). Although these values are not statistically significantly different (Fischer's exact test , P> 0.1) than the expected 40–47% of the possible neutral sites on the coding region relative to the intron (see Methods ), these estimates tend to or deviate significantly from the ∼ 60% changes on the coding region expected from randomly distributed mutations ( P= 0.054 and 0.018, for D. melanogaster and D. simulans respectively; Fischer's exact test). A similar scenario is found in species of the yakuba/erecta clade, in which only 16.7% (8/48) of the DNA sequence variation found in the surveyed RFeSP loci of these species clusters outside intron2 ( Supplementary Fig. S1 ), which departs significantly from the ∼ 60% expected from randomly distributed mutations and the 40–46% expected from neutral site mutations (Fischer's exact test, P< 0.001 and P= 0.001, respectively). These results strongly suggest that RFeSP has been continuously under purifying selection since D. melanogaster and yakuba/erecta clade species last shared a common ancestor. d N /d S analyses of RFeSP -coding region sequences obtained from a variety of key Drosophila taxa further suggested that negative selection was active on the RFeSP locus since all Old world Sophophora flies last shared a common ancestor 25–55 MY ago (MYA) [19] , [20] or earlier ( Fig. 2b ). Importantly, synteny at this chromosomal region has been maintained since D. melanogaster and D. grimshawi last shared a common ancestor about 40–60 MYA [19] , [20] , strongly suggesting that we have followed the evolution of RFeSP sequences originating from the same chromosomal context ( Supplementary Fig. S5 ). The repeated elimination of deleterious alleles from RFeSP loci in D. melanogster ancestors by negative selection was important for the emergence of RFeSP-RA . This imposed a strong bias on the mutations that could accumulate through time on RFeSP , significantly influencing the alternative reading frames, one of which would harbour the future coding sequence of RFeSP-RA ( Fig. 3a ). For instance, the product of the RFeSP-RA transcript could not have been created by the intron2b Δ 62 deletion if there were premature translation termination codons (PTCs) in the alternative reading frame downstream of the ancestral intron2b allele. Indeed, two independent conservative (synonymous) changes were found in the RFeSP-RB mRNA isoform that eliminated two cryptic PTCs ( Fig. 3b ) roughly between 15–20 and 30–60 MYA, respectively [19] , [20] . Hence, the removal of the cryptic PTCs became fixed before the intron2b Δ 62 deletion or even before the intron2 divergence into intron2a and intron2b alleles ( Fig. 3b ). The only cryptic in-frame-PTCs remaining after these fixations were those within the intron2b intron, which were removed in one step by the intron2b Δ 62 deletion. Considering that these changes happened in the context of low d N /d S levels, these conservative changes are strong evidence that the future sequence of RFeSP-RA was a by-product of purifying selection on RFeSP ancestors. 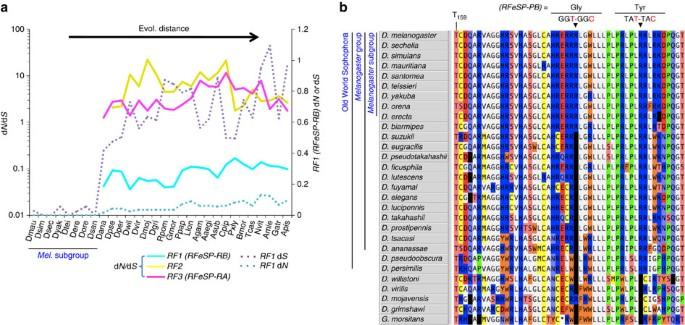Figure 3: Strong negative selection on theRFeSPlocus affected the future coding sequence ofNoble. (a) Ratios of nonsynonymous to synonymous substitutions rates (dN/dS) calculated in the three possible reading frames (RF1–3) of the third exon ofD. melanogaster(Canton-S)RFeSPagainst other taxa. dS(violet dashed lines) and dN(light blue dashed lines) values on theRF1frame are also shown on the scale to the right. Taxa:Drosophila mauritiana(Dmau),D. simulans(Dsim),D. sechellia(Dsec),D. yakuba(Dyak),D. teissieri(Dtei),D. erecta(Dere),D. orena(Dore), D.santomea(Dsan),D. ananassae(Dana),D. pseudoobscura(Dpse),D. persimilis(Dper),D. willistoni(Dwil),D. virilis(Dvir),D. mojavensis(Dmoj),D. grimshawi(Dgri),Rhagoletis pomonella(Rpom),Glossina morsitans(Gmor),Phlebotomus papatasi(Ppap),Lutzomyia longipalpis(Llon),Anopheles gambiae(Agam),Aedes aegypti(Aaeg),Armigeres subalbatus(Asub),Culex pipiens(Cpip),Plutella xylostella(Pxyl),Bombyx mori(Bmor),Tribolium castaneum(Tcas),Nasonia vitripennis(Nvit),Apis mellifera(Amie),Graphocephala atropunctata(Gatr) andAcyrthopsiphon pisum(Apis). (b) Alignment of a C-terminal fragment of the RFeSP-PA protein with the third alternative reading frame starting from the first aa in the third exon of theRFeSPgene of several species. Two cryptic opal PTCs in the third alternative reading frame were transformed into 'CGA' arginine codons (arrowheads) about 15 and 50 MYA, following the divergence of themelanogastersubgroup from othermelanogastergroup species (althoughD. biarmipeshas also lost this PTC), and themelanogastergroup from thewillistonigroup. These changes were a GGT to GGC (maintaining a Gly185in RFeSP-PB) and TAT to TAC (maintaining Tyr199in RFeSP-PB). TheRFeSP-RBisoform without these two PTCs in the alternative reading frame has been maintained for several MY in themelanogastersubgroup, with the exception ofD. erectathat acquired ade novoPTC at a novel position via a GGA to GGT conservative transition (maintaining Gly202in RFeSP-PB). Amino acids are labelled according to their chemical type: acidic (DE), red; hydrophobic (AGILV), white; amido (NQ), light blue; aromatic (FWY), orange; basic (RHK), dark blue; hydroxyl (ST), pink; proline (P), green; sulphur (CM), yellow; and STOP codon, black. Figure 3: Strong negative selection on the RFeSP locus affected the future coding sequence of Noble . ( a ) Ratios of nonsynonymous to synonymous substitutions rates (d N /d S ) calculated in the three possible reading frames (RF1–3) of the third exon of D. melanogaster (Canton-S) RFeSP against other taxa. d S (violet dashed lines) and d N (light blue dashed lines) values on the RF1 frame are also shown on the scale to the right. Taxa: Drosophila mauritiana (Dmau), D. simulans (Dsim), D. sechellia (Dsec), D. yakuba (Dyak), D. teissieri (Dtei), D. erecta (Dere), D. orena (Dore), D. santomea (Dsan), D. ananassae (Dana), D. pseudoobscura (Dpse), D. persimilis (Dper), D. willistoni (Dwil), D. virilis (Dvir), D. mojavensis (Dmoj), D. grimshawi (Dgri), Rhagoletis pomonella (Rpom), Glossina morsitans (Gmor), Phlebotomus papatasi (Ppap), Lutzomyia longipalpis (Llon), Anopheles gambiae (Agam), Aedes aegypti (Aaeg), Armigeres subalbatus (Asub), Culex pipiens (Cpip), Plutella xylostella (Pxyl), Bombyx mori (Bmor), Tribolium castaneum (Tcas), Nasonia vitripennis (Nvit), Apis mellifera (Amie), Graphocephala atropunctata (Gatr) and Acyrthopsiphon pisum (Apis). ( b ) Alignment of a C-terminal fragment of the RFeSP-PA protein with the third alternative reading frame starting from the first aa in the third exon of the RFeSP gene of several species. Two cryptic opal PTCs in the third alternative reading frame were transformed into 'CGA' arginine codons (arrowheads) about 15 and 50 MYA, following the divergence of the melanogaster subgroup from other melanogaster group species (although D. biarmipes has also lost this PTC), and the melanogaster group from the willistoni group. These changes were a GGT to GGC (maintaining a Gly 185 in RFeSP-PB) and TAT to TAC (maintaining Tyr 199 in RFeSP-PB). The RFeSP-RB isoform without these two PTCs in the alternative reading frame has been maintained for several MY in the melanogaster subgroup, with the exception of D. erecta that acquired a de novo PTC at a novel position via a GGA to GGT conservative transition (maintaining Gly 202 in RFeSP-PB). Amino acids are labelled according to their chemical type: acidic (DE), red; hydrophobic (AGILV), white; amido (NQ), light blue; aromatic (FWY), orange; basic (RHK), dark blue; hydroxyl (ST), pink; proline (P), green; sulphur (CM), yellow; and STOP codon, black. Full size image Next, we ruled out that chance alone could account for the fixation of the PTC-losses during the evolution of the RFeSP-RA reading frame. The reduced amount of nucleotide diversity in coding regions of RFeSP compared with its adjacent intron2 had already provided hints of mutational bias on the coding region ( Fig. 2a ; Supplementary Fig. S1 ). A detailed survey of 222 bp of the third exon of RFeSP-RB (from which >70% of the novel coding region of RFeSP-RA originated; Supplementary Table S3 ) showed that the loss of the PTCs during the evolution of RFeSP-RA could have followed trends in codon usage bias during the evolution of the melanogaster group (for example, one PTC was removed while the Tyr codon preference switched from TAT to TAC in Old World sophophorans ( Supplementary Fig. S6 )). This shows that at least one PTC loss was not random, because purifying selection could have been eliminating the mutants with suboptimal codons from populations. Negative selection on RFeSP favours RFeSP-RA persistence Results from the RFeSP codon survey ( Supplementary Table S3 ) also revealed that once RFeSP-RA arose inside the RFeSP locus, it became unlikely that it would be lost by mutation alone. That is, the likelihood that an additional neutral mutation hits any of these 222 nucleotides of RFeSP-RB and at the same time removes RFeSP-RA (by introducing a PTC) is low ( P =0.0015, 0.0165 or 0.0225, if one considers only neutral sites and codon bias, neutral sites and no codon bias, or all possible changes in RFeSP-RB that result in PTCs in RFeSP-RA (even those resulting in aa changes in RFeSP ), respectively; Supplementary Table S3 ). These calculations assume that RFeSP-RA is a neutral or only slightly deleterious feature. If RFeSP-RA has already been (or occasionally becomes) recruited into a functional pathway, it can be predicted that it will itself be subject to natural selection, reducing even further the possibilities of its loss by mutation. The RFeSP intron2 evolved early during Diptera divergence The position of intron2 in the D. melanogaster RFeSP locus (that is, inducing splicing at the aspartic acid, Asp 158 codon of RFeSP ) was essential for the origination of the novel RFeSP-RA transcript by alternative intron retention, so its evolution was investigated further. Molecular phylogenetic analyses of published genomes suggested that an equivalent to the D. melanogaster intron2 had been gained either in an ancestor of the Antliophora (monophyletic group comprising mecopteran lineages, Mecoptera, Siphonaptera and Diptera, which are commonly known as scorpionflies, fleas and true flies, respectively) [27] , or later in a dipteran ancestor, which would conservatively place the intron gain in the Permian (300 MYA) or Jurassic (200 MYA) era, respectively [27] , [28] ( Fig. 4a ). To resolve between these possibilities, sampling was increased across Holometabola (insects with complete metamorphosis), focusing on Antliophora. Results confirmed that apart from the 12-genome reference Drosophila species [29] , the 16 additional Drosophila taxa sequenced in the present study also had the intron2 at Asp 158 . Furthermore, data from non- Drosophila species confirmed that the positioning of intron2 at Asp 158 , or an equivalently positioned aa (referred to as Asp 158 hereafter for simplicity) in other species, was found exclusively in Diptera. Two lower dipteran taxa did not have any intron: the mosquito Culex pipiens and the crane fly Tipula sp. ( Fig. 4a ). Whereas the absence in C. pipiens is attributable to a secondary loss due to the presence of the intron in both Anopheles and Aedes mosquitos, the same is not certain for Tipula sp. ( Supplementary Discussion ). In addition, the sampled dipterans share the secondary loss of a nearby ancient intron localized at arginine Arg 135 , which is 70-nucleotide upstream of the Diptera intron2 at Asp 158 ( Fig. 4a ). The simplest explanation for this finding is that the RFeSP locus suffered a 70-nucleotide upstream (Arg 135 ) intron loss and an independent intron gain at Asp 158 at the time when an ancestor of most or all of the present day Diptera diverged from other Mecopterida (see Fig. 4b for possible scenarios). Therefore, the Asp 158 intron has been stably positioned for at least 200 MY in the lineage that led to D. melanogaster [27] . Intron losses and gains, as well as their persistence, are generally considered to be evolutionarily conservative silent mutations, as they do not necessarily alter the aa-coding sequence [30] . We therefore interpret these results as evidence that stabilizing selection via purifying selection was functioning at the ancestral locus of the D. melanogaster RFeSP locus as the Asp 158 intron was gained. 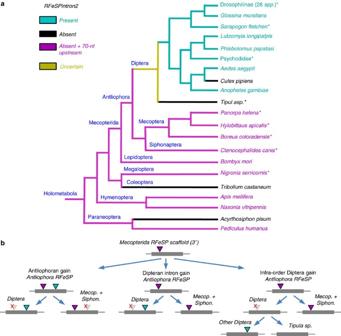Figure 4: TheRFeSP intron2evolved early during Diptera divergence. (a) Scheme ofRFeSP intron2phylogeny regarding its gain at Asp158. The scheme is based on well-established ordinal relationships (for details on the tree construction seeMethods). Asterisks indicate taxa sequenced in this study. Cyan,intron2is present at Asp158or equivalently positioned aa. Magenta,intron2is absent on Asp158but there is an intron 70-nt upstream at Arg135. Black, neither of these introns are found. Dark yellow, uncertain. (b) Three possible scenarios forRFeSP intron2evolution during divergence of Diptera from other Antliophora (Mecoptera (Mecop.) and Siphonaptera (Siphon.)). The grey boxes depict a 3′ stretch (out of scale) of theRFeSPgene scaffold. The magenta arrowhead depicts the ancient 70-nt intron at Arg135. The cyan arrowhead depicts the Asp158intron. A red cross depicts an intron loss event. Figure 4: The RFeSP intron2 evolved early during Diptera divergence. ( a ) Scheme of RFeSP intron2 phylogeny regarding its gain at Asp 158 . The scheme is based on well-established ordinal relationships (for details on the tree construction see Methods ). Asterisks indicate taxa sequenced in this study. Cyan, intron2 is present at Asp 158 or equivalently positioned aa. Magenta, intron2 is absent on Asp 158 but there is an intron 70-nt upstream at Arg 135 . Black, neither of these introns are found. Dark yellow, uncertain. ( b ) Three possible scenarios for RFeSP intron2 evolution during divergence of Diptera from other Antliophora (Mecoptera (Mecop.) and Siphonaptera (Siphon.)). The grey boxes depict a 3′ stretch (out of scale) of the RFeSP gene scaffold. The magenta arrowhead depicts the ancient 70-nt intron at Arg 135 . The cyan arrowhead depicts the Asp 158 intron. A red cross depicts an intron loss event. Full size image Not out of the blue encodes a mitochondrial protein Five key events have been described herein that were essential for the origination of RFeSP-RA (for a scheme with events, see Fig. 5a ). Namely, they were: the positioning of the RFeSP intron2 in an early dipteran ancestor at Asp 158 ; the alternative open-reading frame evolution; the deletions within intron2 ; the dip in intron2b allele diversity; and the reiterated deletion intron2b Δ 62 . A simple interpretation of these successive mutations is that none of them are expected to have been strongly deleterious, or on the other hand to have been a direct cause of positive selection. That RFeSP-RA was generated by the accumulation of neutral or quasi-neutral mutations gives strong support to neutral theories of evolution. 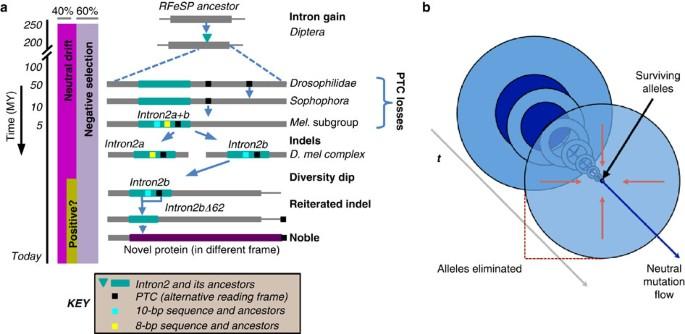Figure 5: Evolutionary steps that generated the novel geneNoble. (a) A series of neutral and quasi-neutral mutations have gradually accumulated for at least 60 MY (since all Drosophilinae shared a common ancestor), or possibly >200 MY (since the gain ofintron2in a dipteran ancestor) of traceable natural selection at theRFeSPlocus inDrosophila melanogaster. The nonrandom accumulation of these mutations recently culminated with the sudden emergence ofRFeSP-RA, here renamedNot out of the blue(Noble). Namely, they were the positioning of the RFeSP intron2 in an early dipteran ancestor at Asp158; the alternative open-reading frame evolution (PTC losses); the deletions withinintron2; the dip inintron2ballele diversity; the reiterated deletionintron2bΔ62; and the generation ofNoble. Left scheme: boxes depict the theoretical proportion of contribution of each evolutionary process: neutral drift, magenta; negative selection, purple. The period when neutral diversity inRFeSPcould have been negatively affected by positive selection atOr22is depicted in yellow. However, it must be stressed that demographical constraints could equally account for this pattern. (b) A scheme showing the fast decay of the probability of a neutral allele suffering iterated neutral mutations. In this space-time scheme, the neutral mutation flow (dark blue, represents 40% of a hypothetical locus—similar to theRFeSPregion we have studied) sinks into an attractor, which is predicted to increase in complexity. The boundaries (limits, light blue and red arrows) are imposed by negative selection. Figure 5: Evolutionary steps that generated the novel gene Noble . ( a ) A series of neutral and quasi-neutral mutations have gradually accumulated for at least 60 MY (since all Drosophilinae shared a common ancestor), or possibly >200 MY (since the gain of intron2 in a dipteran ancestor) of traceable natural selection at the RFeSP locus in Drosophila melanogaster . The nonrandom accumulation of these mutations recently culminated with the sudden emergence of RFeSP-RA , here renamed Not out of the blue ( Noble ). Namely, they were the positioning of the RFeSP intron2 in an early dipteran ancestor at Asp 158 ; the alternative open-reading frame evolution (PTC losses); the deletions within intron2 ; the dip in intron2b allele diversity; the reiterated deletion intron2b Δ 62 ; and the generation of Noble . Left scheme: boxes depict the theoretical proportion of contribution of each evolutionary process: neutral drift, magenta; negative selection, purple. The period when neutral diversity in RFeSP could have been negatively affected by positive selection at Or22 is depicted in yellow. However, it must be stressed that demographical constraints could equally account for this pattern. ( b ) A scheme showing the fast decay of the probability of a neutral allele suffering iterated neutral mutations. In this space-time scheme, the neutral mutation flow (dark blue, represents 40% of a hypothetical locus—similar to the RFeSP region we have studied) sinks into an attractor, which is predicted to increase in complexity. The boundaries (limits, light blue and red arrows) are imposed by negative selection. Full size image A second prediction of the neutral theories of evolution would be that these mutations accumulated stochastically, because of demographical constraints. By following the evolutionary history of the RFeSP locus with high confidence for several MY, we determined that when a productive RFeSP-RA mRNA came about concomitantly with the intron2b Δ 62 deletion, the codons that introduced the novel 102-aa C-terminal part of the RFeSP-PA protein were already set and sculpted by MY of reiterated selected nucleotide sequences that did not affect the RFeSP(-RB) product ( Fig. 5b ). This leads to the conclusion that the emergence of RFeSP-RA by the accumulation of neutral mutations cannot be explained by chance alone; natural selection is required to explain this origination. Hence, the novel RFeSP-RA gene was renamed as Not out of the blue ( Noble ). Noble alludes to the fact that its emergence was influenced by a nonrandom component. Also, it conveys a message about the putative function of its protein product. That is, by lacking a Rieske iron sulphur cluster domain, the Noble protein is likely to be chemically inert or inactive towards oxygen, just like 'Noble' metals (see Fig. 1a ). The respiratory proficient RFeSP-RB gene is hereafter referred to as RFeSP . Next, transgenic and targeted mutagenesis experiments were used to confirm that Noble was indeed translated into a protein in vivo ( Fig. 6 ). In these experiments, the endogenous genome reference strain RFeSP locus (containing intron2b Δ 62 ) was cloned, tagged C-terminally with TagRFP-T and expressed in Drosophila Schneider2 (S2) cells under the control of a Gal4-responsive promoter ( Fig. 6a ). The introduction of a mutation into this construct within the intron that does not affect the coding sequence of RFeSP but results in a Trp 164 to a STOP codon within Noble (resulting in NobleW164STOP ) completely impedes Noble-TagRFP-T production ( Fig. 6a ). The Noble-TagRFP-T gene fusion localized subcellularly to cytoplasmic dots ( Fig. 5b ), which were entirely eliminated in the Trp 164 -STOP mutant, confirming that TagRFP-T fluorescence originates from the full-length Noble protein product fusion ( Fig. 6b ). The complete elimination of splicing from the intron2b Δ 62 locus by targeted mutagenesis (resulting in Noble OPT, for optimal), exclusively produced Noble-TagRFP-T mRNA ( Supplementary Fig. S7 ) and full-length NobleOPT-TagRFP-T protein ( Fig. 6a ). 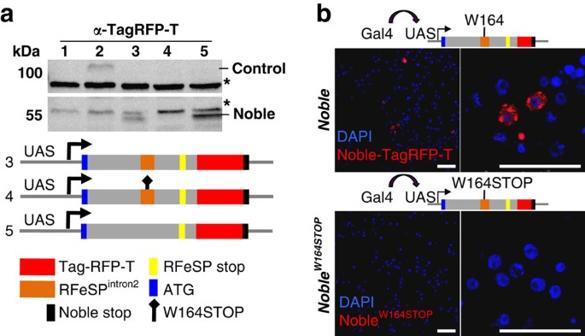Figure 6:Nobleis translated in cultured cells. (a) Western blot ofNoble::TagRFP-Tfusions and mutants with anti-TagRFP-T antibody. Lanes 1–5 pMT-Gal-4. Lane 1: +pUAST(empty vector control). Lane 2: +pUAST-CG9925-TagRFP-T-HA(expected molecular weight (MW) ≈128 kDa), served as a control for the antibody. Lane 3: +pUAST-Noble-TagRFP-T. Lane 4: +pUAST-NobleW164STOP-TagRFP-T. Lane 5: +pUAST-NobleOPT-TagRFP-T. The predicted MW of Noble::TagRFP-T is ≈56 kDa. Asterisks: nonspecific bands. The schematics depicts the pMT-Gal4-dependent pUAST constructs used in the transient transfection experiments performed to obtain theDrosophilaS2 cell lysates loaded in lanes 3–5. Construct 3 ispUAST-Noble-TagRFP-T, in which the endogenous genome reference strainRFeSPlocus (grey) lackingintron1, but containingintron2bΔ62(orange), was cloned and tagged C-terminally with TagRFP-T (red). TheRFeSPgene stop codon is depicted in yellow, whereas theNoble-TagRFP-Tstop is in black. Construct 4 is the same as Constuct 3, but it contains a stop codon instead of Noble-specific amino-acid W164 (black 'stop' sign). Construct 5 is also a modified version of Construct 3, which contains no splice sites forintron2bΔ62at the cost of a Val159Ile mutation. (b) Transiently transfectedDrosophilaS2 cells with theNoble-TagRFP-Tplasmids depicted. Noble-TagRFP-T is in red. 4,6-Diamidino-2-phenylindole (DAPI) is shown in blue on the left. Scale bars, 30 μm. Figure 6: Noble is translated in cultured cells. ( a ) Western blot of Noble::TagRFP-T fusions and mutants with anti-TagRFP-T antibody. Lanes 1–5 pMT-Gal-4. Lane 1: + pUAST (empty vector control). Lane 2: + pUAST-CG9925-TagRFP-T-HA (expected molecular weight (MW) ≈128 kDa), served as a control for the antibody. Lane 3: + pUAST-Noble-TagRFP-T . Lane 4: + pUAST-NobleW164STOP-TagRFP-T . Lane 5: + pUAST-Noble OPT -TagRFP-T . The predicted MW of Noble::TagRFP-T is ≈56 kDa. Asterisks: nonspecific bands. The schematics depicts the pMT-Gal4-dependent pUAST constructs used in the transient transfection experiments performed to obtain the Drosophila S2 cell lysates loaded in lanes 3–5. Construct 3 is pUAST-Noble-TagRFP-T , in which the endogenous genome reference strain RFeSP locus (grey) lacking intron1 , but containing intron2b Δ 62 (orange), was cloned and tagged C-terminally with TagRFP-T (red). The RFeSP gene stop codon is depicted in yellow, whereas the Noble-TagRFP-T stop is in black. Construct 4 is the same as Constuct 3, but it contains a stop codon instead of Noble-specific amino-acid W164 (black 'stop' sign). Construct 5 is also a modified version of Construct 3, which contains no splice sites for intron2b Δ 62 at the cost of a Val159Ile mutation. ( b ) Transiently transfected Drosophila S2 cells with the Noble-TagRFP-T plasmids depicted. Noble-TagRFP-T is in red. 4,6-Diamidino-2-phenylindole (DAPI) is shown in blue on the left. Scale bars, 30 μm. Full size image The subcellular localization of the fusion proteins was determined in vivo with higher resolution in third instar larvae salivary gland cells using well-characterized fluorescently tagged markers. Noble-TagRFP-T tightly associated with mitochondrial markers, but not with other organelles ( Fig. 7 ). In the mitochondria, there was marked heterogeneity on the proportions of Mito-GFP and Noble-TagRFP-T ( Fig. 7a–e ), suggesting mitochondrial dynamics. The same was found in salivary glands of flies expressing Noble-TagRFP-T together with a Mito-YFP reporter ( Fig. 7f–o ), confirming the close association between Noble and mitochondria. Additional experiments with an amino (N)-terminally tagged RFeSP ( intron2b Δ 62 ) locus construct, suggested that Noble, like RFeSP, is N-terminally processed and requires an intact N-terminus to reach the mitochondria ( Supplementary Fig. S8 ). 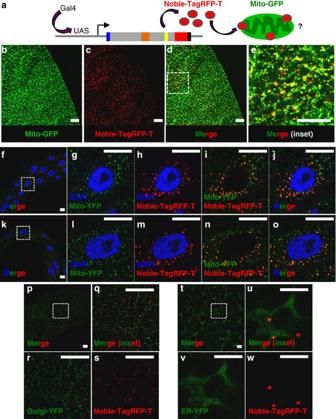Figure 7: Subcellular localization of Noble-TagRFP-T inD. melanogastersalivary gland cellsin vivo. (a)Noble-TagRFP-T(red) was visualized directly together with different subcellular compartment markers fused to YFP or GFP (green) as depicted in this scheme. Subcellular markers are driven by constitutive promoters, which are already highly expressed in the salivary gland precursor cells before the induction ofpUAST-Noble-TagRFP-T. (b) Confocal sections of salivary glands expressing Mito-GFP in green,Noble-TagRFP-Tin red (c). (d) Merge ofbandc. (e) Boxed region fromd. (f) Confocal section of proximal cells of salivary glands expressing Mito-YFP (green) and Noble-TagRFP-T (red). 4,6-Diamidino-2-phenylindole (DAPI) counterstain is in blue. (g–j) Boxed region fromf. (g) DAPI (blue) and Mito-YFP (green). (h) DAPI (blue) and Noble-TagRFP-T (red). (i) Mito-YFP (green) and Noble-TagRFP-T (red). (j) Merge of Mito-YFP (green), Noble-TagRFP-T (red) and DAPI (blue). (k) Confocal section of proximal cells of salivary glands expressing Mito-YFP (green) and Noble-TagRFP-T (red). DAPI counterstain is in blue. (l–o) Boxed region fromk. (l) DAPI (blue) and Mito-YFP (green). (m) DAPI (blue) and Noble-TagRFP-T (red). (n) Mito-YFP (green) and Noble-TagRFP-T (red). (o) Merge of Mito-YFP (green), Noble-TagRFP-T (red) and DAPI (blue). (p) Confocal section of salivary gland cells expressing Golgi-YFP marker (green) and Noble-TagRFP-T (red). Note that the Golgi-YFP localizes to mostly cortical dots in these cells. (q–s) Boxed region fromp. (q) Golgi-YFP (green) and Noble-TagRFP-T (red). (r) Golgi-YFP (green). (s) Noble-TagRFP-T (red). (t) Confocal section of salivary gland cells expressing the endoplasmic reticulum marker (Endo-YFP) in green. Endo-YFP forms a matrix and occupies a significant fraction of the cytoplasm. Large dark roundish areas are secretory vesicles. In cortical areas, Noble-TagRFP-T (red) dots appear squeezed between the reticulum and the vesicles. (u–w) Boxed region fromt. (u) Endo-YFP (green) and Noble-TagRFP-T (red). (v) Endo-YFP (green). (w) Noble-TagRFP-T (red). Scale bars correspond to 30, 20 and 5 μm forb–e,f–sandt–w, respectively. Figure 7: Subcellular localization of Noble-TagRFP-T in D. melanogaster salivary gland cells in vivo . ( a ) Noble-TagRFP-T (red) was visualized directly together with different subcellular compartment markers fused to YFP or GFP (green) as depicted in this scheme. Subcellular markers are driven by constitutive promoters, which are already highly expressed in the salivary gland precursor cells before the induction of pUAST-Noble-TagRFP-T . ( b ) Confocal sections of salivary glands expressing Mito-GFP in green, Noble-TagRFP-T in red ( c ). ( d ) Merge of b and c . ( e ) Boxed region from d . ( f ) Confocal section of proximal cells of salivary glands expressing Mito-YFP (green) and Noble-TagRFP-T (red). 4,6-Diamidino-2-phenylindole (DAPI) counterstain is in blue. ( g – j ) Boxed region from f . ( g ) DAPI (blue) and Mito-YFP (green). ( h ) DAPI (blue) and Noble-TagRFP-T (red). ( i ) Mito-YFP (green) and Noble-TagRFP-T (red). ( j ) Merge of Mito-YFP (green), Noble-TagRFP-T (red) and DAPI (blue). ( k ) Confocal section of proximal cells of salivary glands expressing Mito-YFP (green) and Noble-TagRFP-T (red). DAPI counterstain is in blue. ( l – o ) Boxed region from k . ( l ) DAPI (blue) and Mito-YFP (green). ( m ) DAPI (blue) and Noble-TagRFP-T (red). ( n ) Mito-YFP (green) and Noble-TagRFP-T (red). ( o ) Merge of Mito-YFP (green), Noble-TagRFP-T (red) and DAPI (blue). ( p ) Confocal section of salivary gland cells expressing Golgi-YFP marker (green) and Noble-TagRFP-T (red). Note that the Golgi-YFP localizes to mostly cortical dots in these cells. ( q – s ) Boxed region from p . ( q ) Golgi-YFP (green) and Noble-TagRFP-T (red). ( r ) Golgi-YFP (green). ( s ) Noble-TagRFP-T (red). ( t ) Confocal section of salivary gland cells expressing the endoplasmic reticulum marker (Endo-YFP) in green. Endo-YFP forms a matrix and occupies a significant fraction of the cytoplasm. Large dark roundish areas are secretory vesicles. In cortical areas, Noble-TagRFP-T (red) dots appear squeezed between the reticulum and the vesicles. ( u – w ) Boxed region from t . ( u ) Endo-YFP (green) and Noble-TagRFP-T (red). ( v ) Endo-YFP (green). ( w ) Noble-TagRFP-T (red). Scale bars correspond to 30, 20 and 5 μm for b – e , f – s and t – w , respectively. Full size image Here, a systematic dissection of the evolutionary processes behind the origination of a novel protein-coding sequence has been conducted. Noble's emergence is partially analogous to non-deleterious frameshift-derived gene origins [31] , which have long been hypothesized as an important window for the generation of genetic novelty [32] , [33] . Indeed, similar gene arrangements to the RFeSP/Noble locus have been reported in the literature [31] , [33] , [34] , [35] . In some cases, such as with the relatively new p19ARF tumour suppressor, which is encoded on the alternative reading frame of the more conserved INK4a tumour suppressor [36] , the newest protein component of the locus has clearly integrated into molecular pathways and assumed important functions. In the case of the RFeSP/Noble pair, one can assume that although Noble carries the information and appears to be stable enough to accumulate in the mitochondria, it could not participate positively in mitochondrial respiration because it lacks the smaller iron–sulphur domain, which is found only in RFeSP ( Fig. 1a ). This property hints at a possible regulatory function of Noble on mitochondrial respiration, whereby Noble could directly antagonize RFeSP function. Considering this hypothetical scenario, the finding that Noble emerged by alternative splicing opens up the possibility that the evolution of this protein diversifying process is tightly linked to the abrupt origination of fine-tuned regulatory protein networks. We showed that the 102 codons encoding the C-terminus of Noble emerged de novo in a single step from non-coding DNA by a deletion that induced alternative retention of the second intron of the RFeSP locus. Thus, apart from arising through gradual descent from previously duplicated expressed genetic units, the emergence of Noble demonstrates that new domain-sized protein stretches may form in the absence of expressed and/or functional transitional forms, in what appears to the eyes of the observer as a molecular 'leap'; as if it were out of the blue. Our analyses showed that the non-coding sequences that were used for the generation of Noble had been shaped by the accumulation of nearly neutral mutations at a strongly negatively selected locus, RFeSP , through hundreds of millions of years, probably since RFeSP gained intron2 at Asp 158 very early during Diptera evolution ( Supplementary Discussion ). As neutral or nearly neutral mutations are only a minor subset of the mutations expected to have occurred at this locus, it can be concluded that the origination of Noble was biased by selection, and was therefore not random. This can be contrasted with an eventual origination at a more neutrally evolving locus such as at a pseudogene or duplicated gene, in which most mutations (at least initially for the latter) [37] should have an equal probability of fixation. The mechanisms behind the generation of Noble can explain how a locus can paradoxically diversify and increase the protein repertoire while maintaining ancestral states under strong negative selection without gene duplication, such as during the evolution of alternative splicing. This might provide a rational to explore the different constraints imposed on the evolution of genes by gene duplication and alternative splicing [38] . It is also tempting to suggest that these findings could also shed light onto instances in which de novo protein stretches probably had to originate under highly constrained situations of negative selection, such as during the ab initio protein diversification in early living organisms [39] . Drosophila strains and other insect samples Drosophila flies were raised and crossed at 25 °C. Isofemale lines were established by R.C.W. from wild Drosophila melanogaster lines caught in Ohio, USA. Other insect samples were collected and classified by M.F.W. or A.M.G. and stored in absolute ethanol at −80 °C. A list of the Drosophila lines and the non-Drosophilinae insects used in our study can be found in Supplementary Tables S1 and S4 , respectively. PCR and reverse transcriptase–PCR Drosophila samples were stored in RNAlater TissueProtect Tubes (Qiagen, catalogue #76,154). Genomic DNA was routinely extracted from one male and one female adult per Drosophila line or from parts, or whole individuals, for the other insects using the Dneasy, Blood and Tissue kit (Qiagen, catalogue #69,506). RNA was isolated with Trizol Reagent (Invitrogen, catalogue #15,596-026; larvae and adult flies and insect samples stored in EtOH) or with RNeasy Mini Kit (Qiagen, catalogue #74,106; larvae), and subject to double DNAse digestion: RNAse-free DNase set (Qiagen, catalogue #79,254) and Turbo DNA-free (Ambion, catalogue #AM1907). cDNA was made with SuperScript First-Strand, Synthesis System for RT–PCR (Invitrogen, catalogue #18,080-051). A list with the primers used in this study is provided in Supplementary Table S5 . Sequence analyses and phylogeny PCR products were cleaned with QIAquick PCR purification kit (Qiagen, catalogue #28,106) or if necessary by gel extration using a QIAquick Gel extraction kit (Qiagen, catalogue #28,704). Products from degenerate PCRs were cloned by ligating 1 μl of PCR product with 50 ng of AccepTor Vector, pSTblue-1 vector (Novagen) using a Quick ligation kit (Biolabs, catalogue #M2200S). Subsequently, 1 μl of the ligation reaction was added directly to Novablue Singles Competent Cells (Novagen), which were transformed for 5 min on ice, 30 s at 42 °C and again 2 min on ice. Minipreps were performed with QIAprep Miniprep Kit (Qiagen, catalogue #27,106), and cloned sequences were amplified with standard primers: T7 and SP6. Sequences were read and edited with MacVector. SNAP software was used to calculate d N /d S ratios [21] , [40] . Neutrality tests were performed using all intron2 sequences, or with each intron2 group ( intron2a and intron2b ) alone using Intrapop (by Guillaume Achaz) [41] , where 100,000 coalescence simulations were used to estimate the statistical significance of each test. Deletions counted as a single unique mutational event. For Figure 1d , the RFeSP loci were overlaid onto the well-accepted phylogeny of the melanogaster subgroup [19] , [20] , [29] , [42] , [43] . For Figure 4a , the presence or absence of the dipteran RFeSP intron2 at Asp 158 was overlaid onto a consensus phylogeny extracted from several sources [27] , [28] , [44] , [45] . Tipula sp. was placed basal to both Culicomorpha and Psychodomorpha based on the apparent consensus between morphological and molecular data [27] , [28] , [45] , [46] , [47] . To establish P values for d N /d S estimates we used the p N and p S values (the proportion of nonsynonymous sites and synonymous sites, respectively), and applied Fischer's exact test, considering α =0.05 and p N= p S as the null hypothesis. To estimate the relative amount of possible mutable nucleotides in the RFeSP locus under negative selection, we made two assumptions. First we assumed a conservative value that 80% of intronic sites are not selected for at the nucleotide level. Second, we assumed an equal probability of mutational hits happening between coding and non-coding neutral sites. We then calculated the average and standard deviation of the amount of possible synonymous sites on the surveyed region of RFeSP for 36 Diptera RFeSP homologues. Alternatively, we added to this amount the average proportion of nonsynonymous site substitutions that we found in five basal Diptera relative to D. melanogaster (taxa used, followed by calculated p N: Phlebotomus papatasi 0.072; Lutzomyia longipalpis , 0.089; Anopheles gambiae , 0.059; Aedes aegypti , 0.060; Armigeres subalbatus , 0.0558; and Culex pipens quinquefasciatus , 0.060). We then obtained the average and standard deviation of the latter sums ( p N+average p S for each of the latter five taxa). The difference between these two estimates is to consider as neutral only the synonymous sites or to consider all observed nucleotide substitutions that have happened during the divergence of Diptera neutral, respectively. The latter includes the nonsynonymous changes, which should represent mostly aa changes that do not affect protein function. A list with the database sources of all sequences used in this study can be found in Supplementary Table S6 . Other genome sequences were obtained from the UCSC Genome Browser ( http://genome.ucsc.edu/ ). Recombination rates between RFeSP and Or22 were calculated with the Drosophila melanogaster recombination rate calculator [48] . Nonsense-mediated decay assay in vivo cDNA was produced from mRNA isolated from male larvae carrying different RFeSP intron2 genotypes as depicted in Figure 1c . Upf1 25G is X-linked and eliminates NMD in hemizigous males [49] , as confirmed by the retention of the larger transcript in RpS9 , which served as a positive control [50] . Transgenes and cloning Transgenes are synthetic and fully sequenced ( http://www.geneart.com ). Complete sequences and full descriptions of the transgenes have been deposited in GenBank under references HQ161726-HQ161730. Transgenes consist of the endogenous reference genome strain RFeSP intron2b Δ 62 locus (for these constructs we removed intron1 completely) under the control of a Gal4-responsive promoter. This was either tagged N-terminally or C-terminally with the bright jellyfish green fluorescent protein (GFP) derivative VisGreen [51] or the bright TagRFP-T (a monomeric derivative of eqFP578 from the sea anemone Entacmaea quadricolor ) [52] , respectively. VisGreen should label both proteins encoded by the intron2b Δ 62 locus, RFeSP and Noble, because they share their N-termini. By contrast, TagRFP-T would exclusively label Noble because of its unique C-terminus. All transgenes were cloned into pUAST after digestion with Eco RI/ Not I. S2 cell transfection S2 cells (Invitrogen, catalogue #10,831-014) were maintained in Express Five SFM (Invitrogen, catalogue #10,486-025), supplemented with L -glutamine (from 100× stock, LabClinics, catalogue #M11-004) and antibiotics (from 100× penicillin/streptomycin stock, Sigma, catalogue #P4333-100ML). The cells were grown in an air incubator at 25 °C without CO 2 . For transient transfections, 2 ml of Express Five SFM medium supplemented with L -glutamine 1× containing 8×10 5 Drosophila S2 cells were plated into individual wells of 6-well plates. The DNA for transfection was maxi-prepped (NucleoBond Xtra Maxi kit, Macherey-nagel, catalogue #740414.50). DNA concentrations were determined using the NanoDrop 1,000 spectrophotometer (Thermo Scientific). For individual transfections, we used 2 μg of total DNA including pMT-Gal4 and one of the following plasmids: pUAST empty vector, pUAST-VisGreen-RFeSP/Noble , pUAST-Noble-TagRFP-T , pUAST-NobleW137STOP-TagRFP-T and pUAST-NobleOPT-TagRFP-T. The amount of each plasmid was adjusted to get equimolar concentration. The cells were transfected using Cellfectin II Reagent (Invitrogen, catalogue #10,362-100) according to the manufacturer's protocol using 100 μl Express Five SFM medium supplemented with L -glutamine and 8 μl Cellfectin II Reagent. The metallothionein promoter was induced 24 h after transfection by adding CuSO 4 at 1.4 mM to the cells. Cells were lysed 24 h later (48 h since the start of transfection). Fly transformation Transgenes were injected in w 1118 /yw embryos together with the helper plasmid Δ2–3 using standard P-element-mediated transformation procedures (BestGene). w+ transformant flies were backcrossed again to w 1118 /yw flies and balanced. SDS–polyacrylamide gel electrophoresis and western blotting To prepare whole cell lysates, cells were collected with lysis buffer (50 mM Tris–HCl (pH 8), 150 mM NaCl, 1% NP40, 0.5% sodium deoxycholate, 0,1 % SDS, 1 mM sodium orthovanadate, 1 mM NaF, 2 mM Pefablock, protease inhibitor cocktail tablet (Roche, catalogue #11,836,170,001)), followed by constant agitation for 30 min at 4 °C and centrifugation at 13,000 r.p.m. at 4 °C for 15 min. The soluble fraction was stored at −20 °C. Protein concentrations were determined by the bicinchoninic acid assay (BCA protein assay kit; Pierce, catalogue #23,227). A total of 25 μg of protein were solubilized in sample buffer with β-mercaptoethanol and electrophoresed on denaturing SDS–polyacrylamide gels (10%). The proteins were then transferred to polyvinylidene difluoride membranes (Inmovilon-P Transfer membranes; Millipore, catalogue # IPVH00010), and analysed by western blotting incubating with a 1:3,000 dilution of anti-tRFP at 1 μg μl −1 (Evrogen, catalogue #AB234) or a 1:1,000 dilution of anti-GFP at 2 μg μl −1 (Abcam, catalogue #ab290) overnight at 4 °C. Blots were then washed and incubated with a 1:5,000 dilution of HRP-conjugated anti-rabbit secondary antibody at 10 μg μl −1 (Millipore, catalogue #12–448) for 1 h at room temperature. All antibodies, blockages and washes were performed in 3% non-fat dry milk in 0.1% PBS-Tween-20. Reactive bands were detected with ECL Western Blotting Substrate (Pierce, catalogue #32,209). Immunofluorescence analysis Transfections were performed exactly as described above (see 'S2 Cell Transfection'), except that 1 μg of total DNA was used. Cells on cover slips were fixed with 4% formaldehyde 24 h after the addition of CuSO 4 (48 h since the start of transfection). Cells were then incubated in darkness with 4,6-diamidino-2-phenylindole for 10 min. Slides were mounted in Vectashield (Vector Labs, catalogue #H-1,000) and analysis was performed with an inverted confocal microscope (Laser Scanning confocal Microcope TCS SP2 ADBS, Leica Microsystems, Heidelberg GmbM). For these experiments, transgenic flies carrying either pUAST-VisGreen-RFeSP/Noble or pUAST-Noble-TagRFP-T were crossed to ey-Gal4 (Gal4 under the eyeless enhancer, driving UAS-dependent transcription) in the presence of fluorescent reporters of subcellular organelles [53] , [54] ( Supplementary Table S1 ). Tissue-specific overexpression of the pUAST-VisGreen-RFeSP/Noble or pUAST-Noble-TagRFP-T constructs either alone or together had no detectable effect on developing eye imaginal discs or salivary glands. Wandering third instar larval salivary glands were dissected with PBS and processed as described above. Accession codes: Sequences are deposited in GenBank under accession codes HQ161633 to HQ161730 . How to cite this article: Gontijo, A.M. et al . Intron retention in the Drosophila melanogaster Rieske iron sulphur protein gene generated a new protein. Nat. Commun. 2:323 doi: 10.1038/ncomms1328 (2011).